Amyloid-β nanotubes are associated with prion protein-dependent synaptotoxicity Growing evidence suggests water-soluble, non-fibrillar forms of amyloid-β protein (Aβ) have important roles in Alzheimer’s disease with toxicities mimicked by synthetic Aβ 1–42 . However, no defined toxic structures acting via specific receptors have been identified and roles of proposed receptors, such as prion protein (PrP), remain controversial. Here we quantify binding to PrP of Aβ 1–42 after different durations of aggregation. We show PrP-binding and PrP-dependent inhibition of long-term potentiation (LTP) correlate with the presence of protofibrils. Globular oligomers bind less avidly to PrP and do not inhibit LTP, whereas fibrils inhibit LTP in a PrP-independent manner. That only certain transient Aβ assemblies cause PrP-dependent toxicity explains conflicting reports regarding the involvement of PrP in Aβ-induced impairments. We show that these protofibrils contain a defined nanotubular structure with a previously unidentified triple helical conformation. Blocking the formation of Aβ nanotubes or their interaction with PrP might have a role in treatment of Alzheimer’s disease. Persuasive genetic and biomarker evidence indicates that the amyloid-β protein (Aβ) is the root cause of Alzheimer’s disease (AD) [1] . Like many proteins associated with neurodegenerative conditions, Aβ is prone to self-association and aggregation, and can exist in a large number of different assembly forms. Importantly, certain preparations of synthetic Aβ possess disease-relevant activity, including the ability to disrupt synaptic plasticity in vitro and in vivo . However, the forms of Aβ that mediate this effect and the mechanism by which this occurs remain obscure. For instance, it is not clear if a single oligomeric form of Aβ or a range of Aβ species are required and whether this involves specific cellular receptors [2] , [3] . Most attention is now focused on soluble, oligomeric forms of Aβ, partly because these species are believed to display relatively higher neurotoxicity than either monomeric Aβ or mature amyloid fibrils [2] , [3] . However, soluble oligomers vary in size from dimers through to complex structures containing hundreds of peptide units in different morphologies [4] and a number of receptors for toxic Aβ assemblies have been proposed [5] , [6] , [7] , [8] . Due to difficulties in isolating sufficiently pure native Aβ assemblies from AD brain, synthetic preparations of Aβ that produce specific toxic effects have been extensively studied [2] , [4] , [9] . However, these preparations are heterogeneous, contain an ensemble of different species [2] , [10] and to date no defined Aβ structure has been shown to produce neurotoxicity via a specific receptor. One suggested receptor for toxic Aβ assemblies is prion protein (PrP) [6] , [11] , [12] , [13] , [14] , [15] , [16] , [17] , [18] . Inhibition of long-term potentiation (LTP) [15] and activation of Fyn [19] by AD brain have been shown to be PrP-dependent and mimicked by synthetic Aβ preparations. Aβ assemblies that bind to PrP have also been specifically detected in AD brain [19] , although their size and structure remain unknown. Whilst the ability of certain preparations of Aβ to form an avid complex with PrP has not been disputed [6] , [11] , [14] , [15] , [20] , the relevance of the interaction to AD has been questioned [10] , [11] , [20] , [21] , with one report unable to replicate the PrP-dependent inhibition of LTP by Aβ oligomers [22] . Given these uncertainties, and the heterogeneity and lack of characterization of different synthetic Aβ preparations [10] , it is important to define the active PrP-dependent, PrP-independent and benign species. Such characterization of PrP-dependent toxic Aβ assemblies would then allow a search for these species in vivo and attempts to correlate their presence with AD pathogenesis and progression. Here, we identify protofibrils as the most avid PrP-binding species relative to monomer, globular oligomers or fibrils and show that their presence correlates with PrP-dependent synaptotoxicity. Using electron microscopy (EM), we reveal that these PrP-binding protofibrils are in fact Aβ nanotubes comprising a triple helical structure. We also demonstrate that Aβ fibrils, produced in the same conditions, cause PrP-independent inhibition of LTP. These data resolve some of the conflicting reports regarding PrP-dependent synaptotoxicity of Aβ and identify a novel Aβ structural fingerprint that can now be pursued in AD brain. PrP-binding correlates with presence of Aβ protofibrils Certain preparations of Aβ that contain mixtures of monomer, globular oligomers and protofibrils inhibit LTP in a PrP-dependent manner [6] , [15] . As pure monomeric Aβ 1–42 seems to not inhibit LTP [23] , [24] and does not form a high affinity interaction with PrP [11] , [14] , [15] , we focused our studies on aggregated non-monomeric forms of Aβ 1–42 . To investigate the activity of globular oligomers, protofibrils and mature fibrils we utilized an experimental paradigm that allowed us to temporally resolve pools of Aβ enriched in each of these species ( Fig. 1a–c ), based on a modified version of the Aβ-derived diffusible ligand preparations [6] , [9] , [15] . This involved dissolving hexafluoro-2-propanol (HFIP)-treated Aβ 1–42 in dimethylsulphoxide (DMSO), dilution into phenol red-free Hams-F12 medium, centrifugation and incubation at 22 °C for up to 2 weeks (0–336 h). Samples were aliquoted and snap frozen at regular intervals over the time course. Aβ assembly states were visualized by negative stain EM and relative levels of PrP-binding at 120 nM concentration were determined by an enzyme-linked immunosorbent assay (ELISA)-based protocol detected by dissociation-enhanced lanthanide fluorescent immunoassay (DELFIA) [25] ( Fig. 1d ). The concentration-dependent binding seems to conform to a non-cooperative Langmuir-type isotherm with occupancy increasing from 10 to 90% over a 100-fold concentration range [15] . However, because of uncertainty of the valency of the interactions [15] and because Aβ appears to irreversibly bind to PrP [14] , true equilibrium dissociation constants cannot be determined. Nevertheless, at Aβ concentrations where nonspecific binding is absent and binding occupancy is below 90%, relative estimates of binding can be made. The nanomolar sensitivity of DELFIA gives an advantage over other techniques, such as surface plasmon resonance, electron paramagnetic resonance or NMR that probe the Aβ:PrP interaction at micromolar concentrations, so may not identify subtle differences in binding seen at lower, more physiologically relevant concentrations. 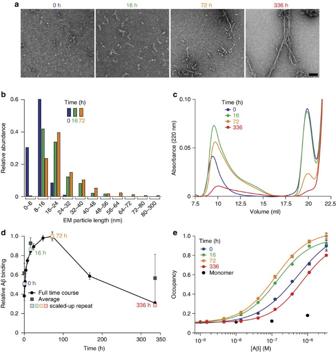Figure 1: Time-dependent aggregation of Ab1–42and binding to PrP. Disaggregated films of Aβ1–42were dissolved in DMSO and Ham’s F12 media, vortexed and centrifuged before incubating at 22 °C for different periods of time without agitation. (a) Representative images of aggregated Aβ assemblies seen by negative stain EM at 0 (blue), 16 (green), 72 (orange) and 336 h (red) with a scale bar of 50 nm. (b) Measurement of the longest dimension of aggregated Aβ assemblies seen by negative stain EM on a carbon-coated film at 0 (blue), 16 (green) and 72 h (orange). Lengths could not reliably be measured for aggregated Aβ assemblies seen at 336 h. (c) Size-exclusion chromatography (SEC) analysis of Aβ assemblies at 0 (blue), 16 (green), 72 (orange) and 336 h (red) in PBS. Although the depletion of monomer can be observed by absorbance, the size of the oligomer peaks and the monomer/oligomer ratio cannot be quantified by absorbance due to a disproportional increase in the apparent oligomer absorbance, possibly due to light scattering or an increased extinction coefficient in the oligomer state. (d) Relative binding of 120 nM Aβ to huPrP detected by DELFIA for the initial time course (black), a scaled-up repeat time course used for further characterization including LTP experiments (coloured) and the average of 11 separate time courses (grey) (n=3, error bars show s.d.). All individual time courses are scaled to the maximum binding sample within that set. A magnified version showing the early time point is shown inSupplementary Fig. S2a. (e) Titration of the relative quantities of PrP-binding Aβ assemblies at 0 (blue), 16 (green), 72 (orange), 336 h (red) and SEC-purified monomer (black) relative to starting concentration of Aβ monomer (n=3, error bars show s.d.). Figure 1: Time-dependent aggregation of Ab 1–42 and binding to PrP. Disaggregated films of Aβ 1–42 were dissolved in DMSO and Ham’s F12 media, vortexed and centrifuged before incubating at 22 °C for different periods of time without agitation. ( a ) Representative images of aggregated Aβ assemblies seen by negative stain EM at 0 (blue), 16 (green), 72 (orange) and 336 h (red) with a scale bar of 50 nm. ( b ) Measurement of the longest dimension of aggregated Aβ assemblies seen by negative stain EM on a carbon-coated film at 0 (blue), 16 (green) and 72 h (orange). Lengths could not reliably be measured for aggregated Aβ assemblies seen at 336 h. ( c ) Size-exclusion chromatography (SEC) analysis of Aβ assemblies at 0 (blue), 16 (green), 72 (orange) and 336 h (red) in PBS. Although the depletion of monomer can be observed by absorbance, the size of the oligomer peaks and the monomer/oligomer ratio cannot be quantified by absorbance due to a disproportional increase in the apparent oligomer absorbance, possibly due to light scattering or an increased extinction coefficient in the oligomer state. ( d ) Relative binding of 120 nM Aβ to huPrP detected by DELFIA for the initial time course (black), a scaled-up repeat time course used for further characterization including LTP experiments (coloured) and the average of 11 separate time courses (grey) ( n =3, error bars show s.d.). All individual time courses are scaled to the maximum binding sample within that set. A magnified version showing the early time point is shown in Supplementary Fig. S2a . ( e ) Titration of the relative quantities of PrP-binding Aβ assemblies at 0 (blue), 16 (green), 72 (orange), 336 h (red) and SEC-purified monomer (black) relative to starting concentration of Aβ monomer ( n =3, error bars show s.d.). Full size image Freshly dissolved Aβ 1–42 ( t =0 h) contained small globular assemblies (11±4 nm) and Aβ monomer ( Fig. 1a–c ) and bound only weakly to PrP. Globular assemblies visualized by atomic force microscopy and prepared in phosphate buffer have previously been shown to bind to PrP by surface plasmon resonance, but the interaction did not saturate by 2 μM, suggesting the interaction may be relatively weak [14] . However, on incubation Aβ readily assembled to form protofibrils 20–200 nm in length ( Fig. 1a–c ) and Aβ in these solutions bound more avidly to PrP ( Fig. 1d ). At later times, when the number of protofibrils had decreased and fibrils predominated, PrP-binding activity declined ( Fig. 1d ). The low binding at 0 and 336 h was still significantly higher than background monomer binding [15] suggesting that these preparations contained some PrP-binding assemblies. Aliquoted samples could be defrosted and tested many weeks apart or diluted and left for 24 h at room temperature without changing the PrP-binding profile ( Supplementary Fig. S1 ). A large-scale repeat of four key time points (0, 16, 72 and 336 h) demonstrated that the trend of low initial binding, rapid increase, a plateau then decrease was qualitatively reproducible ( Fig. 1d ) and not saturated at the nanomolar concentrations used for comparison ( Fig. 1e ). This also confirmed that the PrP-binding and presence of protofibrils remained relatively stable between 16 and 72 h. The retention of higher levels of PrP-binding by some samples incubated for 336 h was consistently associated with presence of short protofibrils and globular structures in those preparations ( Supplementary Fig. S2b–d ). This suggested that protofibrils, rather than monomer or mature fibrils, were the Aβ species that bound most avidly to PrP. The N1 fragment of PrP (23–111) contains the same two Aβ-binding sites as full length PrP [14] , [15] , and has been shown to bind both synthetic and AD brain-derived Aβ oligomers [19] , [26] . When we investigated the binding of Aβ to N1 we found that N1 bound protofibrils to a similar degree as full length PrP, but with greater selectivity ( Supplementary Fig. S3a ) and that the presence of oligomers longer than 20 nm in length best correlated with binding ( Supplementary Fig. S3b ). The repeat preparation showed a similar PrP-binding profile to the initial experiment with the same evolution from globular assemblies to protofibrils then fibrils ( Fig. 1a ). Surface-enhanced laser desorption/ionization-time of flight (SELDI-TOF) mass spectrometry ( Supplementary Fig. S4a ) confirmed that the change in binding was not caused by peptide degradation or modification, SDS–polyacrylamide gel electrophoresis (SDS–PAGE) ( Supplementary Fig. S4b ) showed that most of the peptide remained soluble in SDS up to 72 h, and reactivity with conformation-specific A11 and OC antibodies [27] , [28] suggested that all samples contained ‘fibrillar oligomers’ ( Supplementary Fig. S4c ) that have been shown to have cross-β structure [29] . The level of OC immunoreactivity in DELFIA correlated with total Aβ observed using 6E10, suggesting that the majority of Aβ-binding was in an OC-reactive conformation ( Supplementary Fig. S4d,e ). In contrast, A11 interacted with the high-density PrP [28] saturated on the surface of the plate, but showed no change in signal on addition of any Aβ. Size-exclusion chromatography showed the conversion of monomer to oligomer and then loss of buffer-soluble material ( Fig. 1c ) that is most likely due to precipitation or interaction with the column. The identity of monomeric Aβ was confirmed by static light scattering (molecular weight=4,500±400, Supplementary Fig. S5a ) with a retention time indistinguishable from NaOH-solublized Aβ. The species present at 16 and 72 h, eluting between 10 and 15 ml ( Fig. 1c ), contained protofibrils ( Fig. 1a and Supplementary Fig. S5b ) with molecular masses (estimated by static light scattering) from 10 5 to 10 6 ( Supplementary Fig. S5a ). Some aggregated and fibrillar material was seen between 9 and 10 ml ( Supplementary Fig. S5a,b ). Given that at 0 h Aβ had already formed small oligomeric species, and as it has previously been demonstrated that monomeric Aβ does not interact with PrP in the low nanomolar range [6] , [11] , [14] , [15] , we investigated if the smallest possible Aβ oligomer—a dimer—could bind to PrP. To do this, we used Aβ 1–40 in which Ser26 was substituted with cysteine and the monomers oxidatively crosslinked to produce dimers ((Aβ 1–40 S26C) 2 )( Supplementary Fig. S6a ). Authentic (Aβ 1–40 S26C) 2 showed little interaction with PrP below micromolar concentrations where binding to PrP becomes nonspecific ( Supplementary Fig. S6b ), whereas (Aβ 1–40 S26C) 2 exchanged into PBS readily formed larger assemblies that bound to PrP at low nanomolar concentrations ( Supplementary Fig. S6c ). As we have previously shown that (Aβ 1–40 S26C) 2 per se does not block LTP, but protofibrils formed from (Aβ 1–40 S26C) 2 do, and that (Aβ 1–40 S26C) 2 protofibrils transition only very slowly to fibrils [30] , our new PrP-binding data support the conclusion that protofibrils are the major PrP-binding species. Knowing that the Aβ protofibrils bound most avidly to PrP, we expected the presence of these, and not amyloid fibrils or globular oligomers, to correlate with a PrP-dependent form of neurotoxicity [6] , [15] , [31] . Aβ Protofibrils are associated with PrP-dependent toxicity To explore the relationship between PrP-binding and Aβ-toxicity, we tested the ability of four temporally resolved Aβ populations to block LTP ( Fig. 2 ). Freshly dissolved Aβ (t=0) contains monomer and globular assemblies, bound weakly to PrP and failed to inhibit LTP, suggesting these were not the synaptotoxic assemblies responsible for PrP-dependent toxicity. Although globular Aβ assemblies have previously been reported to bind to PrP, their inhibitory effect on LTP was not established [14] . In preparations where Aβ protofibrils predominate (16 and 72 h), LTP was significantly reduced compared with buffer controls, demonstrating that Aβ preparations rich in protofibrils block LTP. Samples that contained mostly mature fibrils (336 h) also significantly inhibited LTP [32] , but not to a significantly greater extent than the 16 or 72 h samples. As this batch of fibrils only very weakly bound to PrP, including when binding experiments were performed in artificial cerebrospinal fluid (ACSF) ( Supplementary Fig. S7a,b ), this observation suggested that fibrillar Aβ may inhibit LTP through a PrP-independent mechanism. It has previously been demonstrated that the plasticity-disrupting activity of Aβ samples from the 16-h time point requires expression of PrP [6] , [15] . Samples of Aβ incubated for 72 h, which contain much lower monomer concentrations, are also rich in protofibrils and bind avidly to PrP indicating that they might inhibit LTP in a PrP-dependent manner ( Fig. 1 and Supplementary Fig. S3 ). Therefore, we sought to confirm if differentially aggregated Aβ samples could inhibit LTP through distinct mechanisms with different PrP-dependencies. 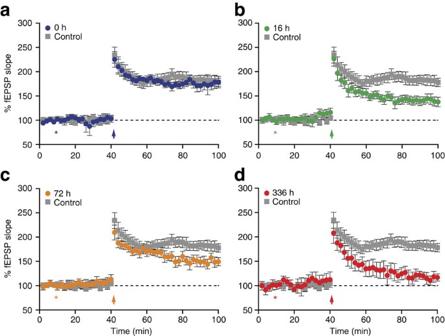Figure 2: Inhibition of LTP induced by different preparations of Ab1–42. Field EPSPs were recorded from the CA1 region of the hippocampus in all cases.P-values were calculated using one-way analysis of variance (ANOVA) and the Tukey–Kramerpost hoctest. Extracellular recordings from C57Bl/6J mice show stable LTP measured up to 1 h post theta burst (grey squares, 179±8%,n=8). Pretreatment of the slices with differentially aggregated Aβ (Fig. 1) for 30 min prior to theta burst showed different effects. (a) Pretreatment with 0-h incubated Aβ did not inhibit LTP (blue, 176±8%,n=6). (b) Pretreatment with 16-h incubated Aβ inhibited LTP (green, 138±9%,P<0.01,n=6). (c) Pretreatment with 72-h incubated Aβ inhibited LTP (orange, 149±9%,P<0.05,n=6). (d) Pretreatment with 336-h incubated Aβ inhibited LTP (red, 122±8%,P<0.01,n=5). No significant differences were observed between the levels of inhibition by the 16, 72 or 336 h time points (error bars show s.e.m.). Figure 2: Inhibition of LTP induced by different preparations of Ab 1–42 . Field EPSPs were recorded from the CA1 region of the hippocampus in all cases. P -values were calculated using one-way analysis of variance (ANOVA) and the Tukey–Kramer post hoc test. Extracellular recordings from C57Bl/6J mice show stable LTP measured up to 1 h post theta burst (grey squares, 179±8%, n =8). Pretreatment of the slices with differentially aggregated Aβ ( Fig. 1 ) for 30 min prior to theta burst showed different effects. ( a ) Pretreatment with 0-h incubated Aβ did not inhibit LTP (blue, 176±8%, n =6). ( b ) Pretreatment with 16-h incubated Aβ inhibited LTP (green, 138±9%, P <0.01, n =6). ( c ) Pretreatment with 72-h incubated Aβ inhibited LTP (orange, 149±9%, P <0.05, n =6). ( d ) Pretreatment with 336-h incubated Aβ inhibited LTP (red, 122±8%, P <0.01, n =5). No significant differences were observed between the levels of inhibition by the 16, 72 or 336 h time points (error bars show s.e.m.). Full size image Using a separate batch of Aβ incubated for 72 h that was rich in protofibrils ( Fig. 3a ), we investigated the effects of this preparation on LTP in hippocampal slices from wild-type and Prnp o/o C57Bl/6J mice. This batch fully inhibited LTP in wild-type mice but had no effect in PrP knock-out mice ( Fig. 3b ). Therefore, both the 16 and 72 h samples contain protofibrils and require expression of PrP to inhibit LTP. In contrast, a batch of fibrillar Aβ blocked LTP in both Prnp o/o and wild-type animals ( Fig. 3c,d ) suggesting that it induces synaptotoxicity through a PrP-independent mechanism. Although LTP can be inhibited to a similar extent by Aβ protofibrils and fibrils, only protofibrillar synaptotoxicity is reversed by PrP ablation. Thus, distinct assemblies appear to elicit toxicity through different pathways with PrP involved in at least one of these—that evoked by protofibrils. PrP does not simply sensitize neurones equally to all forms of Aβ toxicity. These results imply that conflicting reports regarding the required expression of PrP for Aβ synaptotoxicity may be explained due to some investigators using samples contaminated with fibrillar Aβ. Indeed it is noteworthy that centrifugation at 16,100 g for 20 min failed to sediment all fibrillar species, suggesting that oligomer preparations could become contaminated with fibrillar Aβ ( Supplementary Fig. S7c ). We recommend that in future experiments, each aggregated Aβ preparation should be fully characterized to test for contaminating assemblies that may alter their biological activity or specificity. 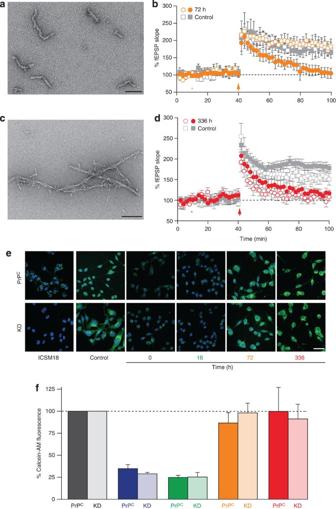Figure 3: PrP-dependence of protofibrillar and fibrillar Aβ assemblies. (a) Representative EM images of 72-h incubated Aβ used inb(scale bar, 50 nm). (b) Comparison of LTP from wild-type (filled symbols) and PrPo/o(hollow symbols) C57Bl/6J mice in the presence (orange symbols) and absence (grey symbols) of 72-h incubated Aβ. LTP from wild-type C57Bl/6J mice in the presence (filled orange circles, 171±16%,n=5) and absence (filled grey squares, 104±14%,n=5) of 72-h incubated Aβ were significantly different (P<0.05), whereas LTP from PrPo/oC57Bl/6J mice in the presence (hollow orange circles, 175±16%,n=5) and absence (hollow grey squares, 181±19%,n=5) of 72-h incubated Aβ show no significant difference. Field EPSPs were recorded from the CA1 region of the hippocampus in all cases.P-values forbanddwere calculated using one-way analysis of variance (ANOVA) and the Tukey–Kramerpost hoctest (error bars show s.e.m.). (c) Representative EM images of fibrillar Aβ used ind(scale bar, 100 nm). (d) Overlay of wild-type (filled symbols also shown inFig. 2d) and PrPo/o(hollow symbols) C57Bl/6J mice in the presence (red symbols) and absence (grey symbols) of fibrillar Aβ. Pretreatment with 336-h incubated Aβ also inhibited LTP in PrPo/oC57Bl/6J mice (hollow red circles, 105±10%,P<0.01,n=5) compared with 336-h incubated buffer (hollow grey squares, 156±13%,n=5) suggesting the effect is PrP-independent. No significant differences were observed between the levels of LTP induced in wild-type and PrPo/omice (error bars show s.e.m.). (e) Representative images of calcein-AM leakage in untreated controls (control; grey) or cells exposed to Aβ aggregated for 0 (purple), 16 (green), 72 (orange) and 336 h (red) for 1 h with a scale bar of 50 μm. (f) Calcein-AM leakage in untreated controls (control; grey) or cells exposed to Aβ aggregated for 0 (blue), 16 (green), 72 (orange) and 336 h (red) used inFigs 1and2for 1 h. PrP-overexpressing and knockdown cells (KD) are represented using darker and lighter shades, respectively. Calcein-AM fluorescence was normalized by cell number and calculated with respect to untreated controls, where fluorescence was taken to be 100% (n=3, error bars show s.e.m.). Figure 3: PrP-dependence of protofibrillar and fibrillar Aβ assemblies. ( a ) Representative EM images of 72-h incubated Aβ used in b (scale bar, 50 nm). ( b ) Comparison of LTP from wild-type (filled symbols) and PrP o/o (hollow symbols) C57Bl/6J mice in the presence (orange symbols) and absence (grey symbols) of 72-h incubated Aβ. LTP from wild-type C57Bl/6J mice in the presence (filled orange circles, 171±16%, n =5) and absence (filled grey squares, 104±14%, n =5) of 72-h incubated Aβ were significantly different ( P <0.05), whereas LTP from PrP o/o C57Bl/6J mice in the presence (hollow orange circles, 175±16%, n =5) and absence (hollow grey squares, 181±19%, n =5) of 72-h incubated Aβ show no significant difference. Field EPSPs were recorded from the CA1 region of the hippocampus in all cases. P -values for b and d were calculated using one-way analysis of variance (ANOVA) and the Tukey–Kramer post hoc test (error bars show s.e.m.). ( c ) Representative EM images of fibrillar Aβ used in d (scale bar, 100 nm). ( d ) Overlay of wild-type (filled symbols also shown in Fig. 2d ) and PrP o/o (hollow symbols) C57Bl/6J mice in the presence (red symbols) and absence (grey symbols) of fibrillar Aβ. Pretreatment with 336-h incubated Aβ also inhibited LTP in PrP o/o C57Bl/6J mice (hollow red circles, 105±10%, P <0.01, n =5) compared with 336-h incubated buffer (hollow grey squares, 156±13%, n =5) suggesting the effect is PrP-independent. No significant differences were observed between the levels of LTP induced in wild-type and PrP o/o mice (error bars show s.e.m.). ( e ) Representative images of calcein-AM leakage in untreated controls (control; grey) or cells exposed to Aβ aggregated for 0 (purple), 16 (green), 72 (orange) and 336 h (red) for 1 h with a scale bar of 50 μm. ( f ) Calcein-AM leakage in untreated controls (control; grey) or cells exposed to Aβ aggregated for 0 (blue), 16 (green), 72 (orange) and 336 h (red) used in Figs 1 and 2 for 1 h. PrP-overexpressing and knockdown cells (KD) are represented using darker and lighter shades, respectively. Calcein-AM fluorescence was normalized by cell number and calculated with respect to untreated controls, where fluorescence was taken to be 100% ( n =3, error bars show s.e.m.). Full size image As we did not expect all Aβ toxicity to be governed by PrP, we tested the PrP-dependence of cell membrane leakage, which has previously been suggested to be caused by direct binding to the lipid bilayer rather than by a receptor-mediated mechanism [33] . The induction of membrane leakage was PrP-independent and did not correlate with the presence of Aβ protofibrils or inhibition of LTP ( Fig. 3e,f ), consistent with suggestions that this phenomenon may be non-specific [2] and requires the presence of Aβ monomer [34] , [35] . This highlights how different preparations of Aβ can have entirely different toxicities working via different mechanisms and that only some will require specific receptors such as PrP. Ab protofibrils are nanotubes with triple helical structure To investigate the structure of protofibrils that bound to PrP and were present in Aβ preparations showing PrP-dependent toxicity, we performed structural analysis by EM ( Fig. 4a ). Although the extended assemblies are very flexible, they showed signs of repeating substructures. Three-dimensional (3D) analysis by negative stain EM and tomography revealed that the protofibrils are helical tubes ~10 nm in diameter with a repeat of 7.8 nm ( Fig. 4b,d ). Tomographic 3D reconstructions revealed that the surface in contact with the support film was flattened, so that the helical structure was only visible on the free surface, implying that the structure is highly deformable. To get a clearer view of the 3D structure, a single particle data set was collected and short segments of the tubes were extracted, aligned and classified. Many of the class averages showed distinct patterns consistent with a helical repeat ( Fig. 4c ). Using the helical repeat determined from the tomograms, reconstructions of continuous helices were generated from the class averages. These showed consistent features and six of these were aligned and averaged to give the structure shown in Fig. 4e . The map reveals a triple helix of density wound around a hollow core. An Aβ amyloid fibril [36] , Aβ β-arch [37] and the PrP c fold [38] are shown for comparison ( Fig. 4f,g,h ). That an inherently unstructured peptide can form such an elaborate nanostructure is remarkable and could conceivably be the source of the specific, PrP-dependent, toxic activity seen in preparations containing Aβ nanotubes. Analysis by tomography of protofibrils that inhibited LTP in a PrP-dependent manner ( Fig. 3a,b ) confirmed that these assemblies contained similar features, consistent with the nanotube structure ( Fig. 4i ), even after shipping on dry ice. 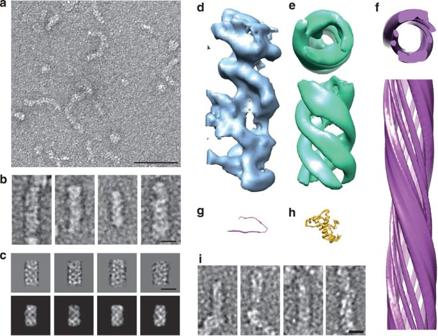Figure 4: EM and tomography reveal a tubular helical structure in protofibrils from the 16 h time point. (a) A representative grid area used to select Aβ assemblies for single particle analysis with a scale bar of 50 nm. (b) Section through reconstructions of four negatively stained Aβ assemblies by electron tomography with a scale bar of 10 nm. Elongated segments of the flexible tubes suggest the presence of ordered substructures. (c) Upper row, averages of classified images of segments of the tubes extracted for single particle analysis, showing distinct repeat patterns with a scale bar of 10 nm. The lower row shows reprojections of the corresponding 3D reconstructions. (d) Isosurface view of a tomography reconstruction showing the helical nature of the tube. The repeat distance is 7.8 nm. (e) Isosurface view of a 3D reconstruction obtained by averaging the structures from six single particle maps, using the pitch repeat of 7.8 nm. The structure shows a triple helical tube (EM Databank accession codeEMD-2433). (f) Isosurface view of a 3D reconstruction of an Aβ amyloid fibril (EM Databank accession codeEMD-5052(ref.36)) has a similar width, but a much longer helical pitch. (g) Ribbon structure of an Aβ in a β-arch conformation from an amyloid-like assembly (PDB code 2LMQ) for a scale comparison. (h) Ribbon structure of the ordered part of PrPc(PDB code 2L39) for comparison. (i) Sections through electron tomography reconstructions of four negatively stained Aβ assemblies incubated for 72 h also suggest the presence of tubes with ordered substructures (scale bar, 10 nm). Figure 4: EM and tomography reveal a tubular helical structure in protofibrils from the 16 h time point. ( a ) A representative grid area used to select Aβ assemblies for single particle analysis with a scale bar of 50 nm. ( b ) Section through reconstructions of four negatively stained Aβ assemblies by electron tomography with a scale bar of 10 nm. Elongated segments of the flexible tubes suggest the presence of ordered substructures. ( c ) Upper row, averages of classified images of segments of the tubes extracted for single particle analysis, showing distinct repeat patterns with a scale bar of 10 nm. The lower row shows reprojections of the corresponding 3D reconstructions. ( d ) Isosurface view of a tomography reconstruction showing the helical nature of the tube. The repeat distance is 7.8 nm. ( e ) Isosurface view of a 3D reconstruction obtained by averaging the structures from six single particle maps, using the pitch repeat of 7.8 nm. The structure shows a triple helical tube (EM Databank accession code EMD-2433 ). ( f ) Isosurface view of a 3D reconstruction of an Aβ amyloid fibril (EM Databank accession code EMD-5052 (ref. 36 )) has a similar width, but a much longer helical pitch. ( g ) Ribbon structure of an Aβ in a β-arch conformation from an amyloid-like assembly (PDB code 2LMQ) for a scale comparison. ( h ) Ribbon structure of the ordered part of PrP c (PDB code 2L39) for comparison. ( i ) Sections through electron tomography reconstructions of four negatively stained Aβ assemblies incubated for 72 h also suggest the presence of tubes with ordered substructures (scale bar, 10 nm). Full size image Elongated or tubular protofibrils have previously been observed by negative stain EM of Aβ assemblies [39] and the residues forming their β-strand structural elements have been identified by NMR [40] , [41] . It is possible that several of these monomer conformers may be present within larger structures such as protofibrils or fibrils [37] , [42] . Hollow structures have been previously described for Aβ and other amyloid fibrils, but the amyloid fibrils are much longer and less flexible, with a helical pitch of 40–60 nm, 4–6 times longer than the pitch of the helical nanotubes [36] ( Fig. 4f ). Such fibrillar structures could also be toxic, although fibrils produced after 2 weeks in our preparations seem to elicit toxicity through an as yet undefined PrP-independent mechanism. Likewise, we show that membrane leakage does not require PrP and the assemblies involved can be distinct from those that cause either PrP-dependent or PrP-independent inhibition of LTP. AD is a clinicopathological syndrome with multiple genetic and environmental factors contributing to its aetiology and rate of progression, and the many cellular and animal models of AD are heterogeneous. As such, it seems implausible that a single receptor molecule could be responsible for all toxicity in all experimental paradigms containing distinct Aβ assemblies, let alone for all clinical and pathological features in the diverse population of AD patients. However, a defined subset of toxic effects may be both specific to a particular receptor and therapeutically targetable, as seems to be the case for PrP-dependent inhibition of synaptic plasticity [6] , [15] , [31] . Indeed, our data demonstrating that protofibril synaptotoxicity requires PrP expression and that water-soluble extracts of AD brain block LTP in a PrP-dependent fashion [15] imply that Aβ nanotubes are also present in human brain and have an important role in disease. With regard to the conflicting results concerning the involvement of PrP in phenotypes reported in amyloid precursor protein transgenic mice, it may be that PrP-dependent [12] , [13] and PrP-independent effects [20] , [21] seen in different animal models of AD could in part be explained by the transitory nature of key Aβ species. The newly discovered order in Aβ nanotubes could have relevance for Aβ toxicity in AD and may help explain apparent inconsistencies regarding the role of PrP in different models of this heterogeneous disease. It will be important to determine if Aβ nanotubes or other recently identified structures [29] , [43] are responsible for the PrP-dependent, synaptic plasticity-impairing effects of ex vivo AD brain extracts [15] . Targeting PrP–Aβ nanotube interactions, for example, with humanized versions of anti-PrP monoclonal antibodies demonstrated to block the Aβ-mediated disruption of synaptic plasticity [15] , may have a role in AD therapeutics. Production of differentially aggregated Ab Aβ 1–42 was synthesized and purified by Dr. James I. Elliott at Yale University (New Haven, CT). The peptide (~1.25 mg) was weighed into a screw-cap 1.5 ml Eppendorf tube, dissolved in ice-cold HFIP to a concentration of 1 mM, sonicated for 10 min, the tube sealed and left to stand at room temperature for 1 h. The solution was then transferred to a 2 ml glass vial and the HFIP evaporated under a stream of dry air/N 2 to produce a clear film. The peptide film was dissolved in anhydrous DMSO with vigorous vortexing for 2 min to produce a 5 mM solution and then diluted to 100 μM in phenol red-free Ham’s F12 medium without L -glutamine (Caisson Labs) and vortexed for 15 s. The sample was transferred to a 2 ml Eppendorf tube, centrifuged at 16,100 g for 5 min to remove any large preformed aggregates and the upper 90% for each solution collected, aliquoted, snap frozen in liquid N 2 and stored at −80 °C. This was considered to be 0 h. For larger time courses, multiple batches were produced and combined at 0 h. Samples were then removed from the freezer and incubated at 22 °C without agitation for between 0 and 336 h before being subaliquoted, snap frozen in liquid N 2 and stored at −80 °C. No further centrifugation was performed at this point. Protein expression and purification Constructs of human PrP were expressed [44] and purified [45] in a similar manner to previously described, but with a second Ni-NTA column after thrombin cleavage. Protein quality was confirmed by SDS–PAGE, matrix-assisted laser desorption/ionization-time of flight (MALDI-TOF) mass spectrometry and circular dichroism spectroscopy. Mass spectrometry Ten microlitres of differentially aggregated Aβ (phenol red-free Ham’s F12 medium, no L -glutamine, 2% DMSO) was applied to an NP20 SELDI-TOF chip (Bio-Rad), incubated for 2 min and removed. The samples were then washed with 2 × 10 μl of mass spectrometry-grade water before the application of a 2,5-dihydroxy benzoic acid film. Samples were run in low mass positive ion mode on a SELDI-TOF ProteinChip Reader PBS-IIC. Dot blot analysis One microlitre of differentially aggregated Aβ (phenol red-free Ham’s F12 medium, no L -glutamine, 2% DMSO) was spotted directly onto nitrocellulose membrane, air dried, blocked with Odyssey Blocking buffer (Licor) for 1 h, then probed with either OC (Millipore) (1:500 dilution), A11 (Millipore) (1:500 dilution) or 6E10 antibody (Covance) (1 μg ml −1 ) in Odyssey Blocking buffer (Licor) for 1 h. OC and A11 were detected with IRDye 800CW goat anti-rabbit IgG antibody, whereas 6E10 was detected with IRDye 800CW goat anti-mouse IgG antibody. The membrane was then dried and visualized using an Odyssey scanner. SDS–PAGE silver staining Ten microlitre aliquots of 100 μM differentially aggregated Aβ (phenol red-free Ham’s F12 medium, no L -glutamine, 2% DMSO) were diluted into sample buffer, boiled, electrophoresed on 16% polyacrylamide tris-tricine gels and visualized by silver staining. Size-exclusion chromatography and multi-angle light scattering Aliquots of differentially aggregated Aβ (phenol red-free Ham’s F12 medium, no L -glutamine, 2% DMSO) of 0.18 or 0.35 ml were injected onto a Superdex 200 10/30 column (GE Healthcare) and eluted with PBS at a flow rate of 0.5 ml min −1 using an Agilent HPLC and peptide elution monitored by absorbance at 220 or 275 nm. Light scattering was performed using a Wyatt DAWN HELEOS II multi-angle light scattering module with Aβ concentrations calculated using the extinction coefficient of tyrosine at 275 nm (1,400 M −1 cm −1 ). (Aβ 1–40 S26C) 2 aliquots of 0.5 ml incubated overnight in 6 M guanidinium chloride were injected onto a Superdex 200 10/30 column and eluted with 25 mM ammonium acetate (pH 8.5) or PBS at a flow rate of 0.5 ml min −1 using an AKTA FPLC and peptide elution monitored by absorbance at 280 nm. Electron microscopy Four microlitre drops of peptide solution were loaded onto negatively glow-discharged copper grids that had been previously coated with a continuous carbon film. Samples were left to adhere for 30 s and excess solution blotted with grade 4 Whatman paper, stained with 2% uranyl acetate (6 μl) for 30 s, blotted and air dried. For single particle reconstruction, low dose images were recorded on an FEI Tecnai T12 electron microscope operating at 120 kV at × 42,986 on Kodak SO-163 film, with a defocus range of 0.7–1 μm. Images were digitized at a step size of 7 μm using a Zeiss SCAI scanner, giving a sampling of 1.63 Å per pixel. Other images were acquired on an FEI Tecnai T10 electron microscope operating at 100 kV and recorded on a 1 k × 1 k charge-coupled device (CCD) camera (Gatan) at a typical magnification of 34,000 with a pixel size of 5.03 Å. Tomography Grids were prepared as described for negative stain analysis. Dual axis tilt series were acquired on an FEI Tecnai F20 microscope operating at 200 kV ( Fig. 4b,d ) or an FEI Tecnai T12 electron microscope operating at 120 kV ( Fig. 4i ). The tilt range was between −68° and +68° with 2° increments and the defocus ranged from 1.5 to 3 μm. Images were either recorded on a 4 k × 4 k CCD camera (Gatan) at a magnification of 38,000 giving a pixel size of 3.92 Å ( Fig. 4b,d ) or on a 1 k × 1 k CCD camera (Gatan) at a magnification of 42,000 with a pixel size of 4.15 Å ( Fig. 4i ). Tomograms were reconstructed from the tilt series with IMOD [46] software using local patch tracking for alignment. From the final tomograms, segments of oligomers showing ordered structural features were extracted and visually inspected in CHIMERA. Volumes that showed strong helical features were converted to SPIDER format and low-pass filtered and masked to remove noise. Single particle reconstruction Defocus parameters for each micrograph were determined with the MRC program CTFFIND3 (ref. 47 ). Micrographs were corrected for the phase reversals of the contrast transfer function using SPIDER [48] and binned to 3.26 Å per pixel before particles (straight segments of the rod-like structures) were manually picked in Boxer [49] and extracted into 80 by 80 pixel boxes. The particles were filtered between 100 and 10 Å and normalized using IMAGIC [50] . Particles were initially aligned to a vertical rectangle and the aligned images were then classified using multivariate statistical analysis (MSA) into classes containing on average 25 images. Classes were manually inspected and ones showing the highest similarity between the individual particles and their corresponding class average were selected for multi-reference alignment (MRA). Following two rounds of MRA/MSA, 3D reconstructions were calculated from the class averages showing the clearest features, using helical symmetry in SPIDER. The helical pitch repeat was estimated by helically averaging the clearest tomogram reconstruction over a range of repeat values and cross-correlating the resulting averages with the unaveraged tomographic reconstruction in CHIMERA. This comparison gave a clear optimum for the helical repeat, at 7.8 nm, and this value was used for helical reconstruction of the single particle class averages. Models from six different class averages, containing a total of 155 segments, were averaged in CHIMERA. As it was not possible to determine a subunit repeat from diffraction patterns of the negatively stained images, probably due to the flexible nature of the helical oligomer, the 3D maps were reconstructed with a subunit repeat of 1 pixel (3.3 Å) to generate continuous helices. Electrophysiology Work with animals was performed under licence granted by the UK Home Office (PPL 70/7274) and conformed to University College London institutional and ARRIVE guidelines. Male, 2–4-month-old C57Bl/6J (Charles River, Margate, UK) or PrP null C57Bl/6J mice (EMMA) were used to study the effects of differentially aggregated Aβ. Mice were anesthetized with isoflurane/O 2 and decapitated. The brain was rapidly removed and immersed in ice-cold sucrose-based artificial cerebrospinal fluid containing 87 mM NaCl, 2.5 mM KCl, 7 mM MgSO 4 , 0.5 mM CaCl 2 , 25 mM NaHCO 3 , 25 mM glucose, 1.25 mM NaH 2 PO 4 and 75 mM sucrose. Parasagital sections (350 μm) were prepared on a Leica VT1000S vibratome using stainless steel razor blades (Campden, Loughborough, UK). Slices were immediately transferred to a holding chamber (BSC-PC, Warner Instruments, Hamden, CT) containing ACSF: 119 mM NaCl, 2.5 mM KCl, 1.3 mM MgSO 4 , 2.5 mM CaCl 2 , 26.2 mM NaHCO 3 , 11 mM glucose and 1.25 mM NaH 2 PO 4 . Circulating ACSF was continuously bubbled with a mixture of 95% O 2 and 5% CO 2 and slices allowed to recover for at least 90 min at room temperature. Extracellular recordings were performed as described previously [15] . Briefly, slices were submerged in a recording chamber and perfused with oxygenated ACSF at a rate of 2–3 ml min −1 and the perfusate warmed to 30 °C. A stainless steel microelectrode (FHC, Bowdoin, USA) was used to stimulate Schaffer collateral fibres, and extracellular field EPSPs were recorded from stratum radiatum of CA1 using a glass microelectrode. EPSPs were recorded using an Axopatch 1D in tandem with a Digidata 1440A digitiser (Axon Instruments). Data were collected using pClamp 10 software and analysed using Clampfit 10.2 (Molecular Devices). For all experiments, test stimuli were given once every 30 s (0.033 Hz), and the stimulus intensity was set to give a baseline fEPSP of 40–50% of the maximal response. A stable baseline was recorded for at least 20 min before application of Aβ. In experiments using differentially aggregated Aβ (stock solutions were diluted 1:200 into ACSF to produce nominal concentrations of 500 nM based on the starting weight of Aβ 1–42 monomer), the sample was added to the perfusate 30 min before induction of LTP. LTP was induced by theta burst stimulation (10 bursts of 4 stimuli at 100 Hz, with an interburst interval of 200 ms) given at baseline intensity. The ACSF was recycled using peristaltic pumps (101 U/R, Watson–Marlow, UK) ensuring that the Aβ was present for the duration of the experiment. LTP is expressed as the mean±s.e.m. % of baseline fEPSP slope. Statistical comparisons used analysis of variance with post hoc Tukey–Kramer test or unpaired Student’s t -test where appropriate. Dissociation-enhanced lanthanide fluorescent immunoassay Fifty microlitres of 1 μM human PrP 23–231 or PrP 23–111 (10 mM sodium carbonate, pH 9.6) was bound to medium binding 96-well white plates (Greiner) with shaking at 400 r.p.m. for 1 h at 37 °C, washed with 3 × 300 μl of PBS (0.05% Tween-20), blocked with 300 μl Superblock (Thermo Scientific) with shaking at 400 r.p.m. at 37 °C for 1 h and washed with 3 × 300 μl of PBS (0.05% Tween-20). Fifty microlitres of different preparations of Aβ 1–42 were incubated in PBS (0.05% Tween-20, 0.1% BSA) or ACSF (see above) for 1 h at 25 °C with shaking at 400 r.p.m. and washed with 3 × 300 μl of PBS (0.1% Tween-20). Aβ was detected by 50 μl of 1 μg ml −1 6E10 in DELFIA assay buffer (PerkinElmer) for 1 h at 25 °C with shaking at 400 r.p.m., washed with 3 × 300 μl of PBS (0.05% Tween-20), incubated for 1 h at 25 °C with shaking at 400 r.p.m. with 300 ng ml −1 of DELFIA Eu-N1 anti-mouse antibody in DELFIA assay buffer (PerkinElmer), washed with 3 × 300 μl of PBS (0.05% Tween-20) before enhancing with 100 μl of DELFIA Enhancement Solution (PerkinElmer) [25] . Alternatively, 1:1,000 OC or A11 (Millipore) were used for detection along with 300 ng ml −1 of DELFIA Eu-N1 anti-rabbit antibody. Plates were scanned for time-resolved fluorescence intensity of the europium probe ( λ ex =320 nm, λ em =615 nm) using a PerkinElmer EnVision plate reader. Apparent XC 50 values were calculated using a 4-parameter XC 50 curve with the maximum plateau signal for a given series used to define full occupancy. Defrosted time course samples that were assayed many weeks apart showed similar binding profiles as did those diluted to 120 nM in PBS (0.05% Tween-20) for 24 h. Cell-based membrane leakage Aβ-induced membrane permeabilization was assessed by monitoring calcein-AM leakage, as previously described [51] . PrP-overexpressing and knockdown murine neuroblastoma (PK1) cells (D-Gen Ltd) [52] were seeded on coverslips overnight and fixed for 30 min with PBS-buffered 4% paraformaldehyde the next day. Cells were then loaded with 3 μM calcein-AM (Invitrogen) for 30 min at 37 °C, washed four times with PBS and subsequently exposed to 500 nM differentially aggregated Aβ for 1 h at 37 °C. Cells were washed four times with PBS, mounted using 4',6-diamidino-2-phenylindole (DAPI)-containing medium (Abcam) and cells were visualized using a Zeiss confocal laser scanning microscope (Carl Zeiss LSM 510). Images were acquired using a Plan-Neofluar 40x/1.3 Oil DIC objective and λ ex =405 nm (DAPI) or 488 nm (calcein-AM), with ImageJ software (NIH) used to quantify images. To detect PrP, cells were seeded on coverslips and fixed as previously described [45] . Cells were then incubated for 1 h at 4 °C with 0.6 μg ml −1 ICSM18 (in PBS), washed four times with PBS, and subsequently incubated for 1 h at 4 °C with 2 μg ml −1 fluorescein-labelled anti-mouse IgG antibody (in PBS). Cells were washed a further four times with PBS, mounted and visualized by confocal microscopy ( λ ex =488 nm for fluorescein). Accession code: The structure of the Aβ nanotube has been deposited in the EM Databank with accession code EMD-2433 . How to cite this article: Nicoll, A. J. et al. Amyloid-β nanotubes are associated with prion protein-dependent synaptotoxicity. Nat. Commun. 4:2416 doi: 10.1038/ncomms3416 (2013).